A walk along DNA using bipedal migration of a dynamic and covalent crosslinker DNA has previously served as an excellent scaffold for molecular transport based on its non-covalent base pairing to assemble both stationary and mobile elements. Use of DNA can now be extended to transport systems based on reversible covalent chemistry. Autonomous and bipedal-like migration of crosslinking within helical DNA is made possible by tandem exchange of a quinone methide intermediate. In this report, net transport is illustrated to proceed over 10 base pairs. This process is driven towards its equilibrium distribution of crosslinks and consumes neither the walker nor the track irreversibly. Successful migration requires an electron-rich quinone methide to promote its regeneration and a continuous array of nucleophilic sites along its DNA track. Accordingly, net migration can be dramatically influenced by the presence of noncanonical structures within duplex DNA as demonstrated with a backbone nick and extrahelical bulge. Developing transportation devices on a molecular scale provides a challenging test of our ability to predict, design and apply non-covalent and covalent forces in complex and dynamic systems. Nucleic acids serve a prominent role in these and related topics involving nanomaterials because of their ready availability and programmable assembly [1] , [2] , [3] . Most examples of transport rely on DNA as both the track and mobile element. Motion is regulated by reversible base pairing in combination with either oligonucleotide displacement or strand hydrolysis as a source of energy. The original two strategies reported in the literature required repeated intervention to drive transport [4] , [5] , but soon an autonomously powered system was created using a DNAzyme [6] . Recent strategies have grown in sophistication to earn the title of a molecular robot [7] and detection has advanced to allow direct observation in real time [8] . Bipedal walking along footholds of complementary strands within arrays of DNA in particular has drawn inspiration from motor proteins such as myosin and kinesin [9] , [10] . In all of the above examples, movement requires infusion of energy or consumption of the track. The use of covalent but reversible bonding for stepwise transfer of a mobile element presents another challenge for expanding the repertoire of molecular transport. Efforts towards this goal are still very much in their infancy and have primarily focused on systems of modest size [11] . Issues to be addressed include the kinetic barriers typically encountered during exchange of covalent bonds, the complex syntheses often required for generating the target molecules and the inherent flexibility of most one dimensional tracks used for guidance. Advances in this topic have directly benefitted from past success in the broader field of dynamic combinatorial chemistry involving reversible covalent forces to assemble new materials and devices from pools of competing subunits [12] , [13] , [14] , [15] , [16] . Only a limited number of covalent bonds have yet demonstrated sufficient reversibility to support these types of applications and most involve exchange through disulfide bonds, iminium ions, hydrazones or boronate complexes [17] . Metal–ligand interactions have also been used for exchange within dynamic mixtures [18] , and a few examples suggest that Michael reactions have a potential for reversible assembly of macromolecules as well [19] , [20] . In particular, a Michael reaction based on α-methylene-4-nitrostyrene was used as the basis for one of the most extensive transfers to date of a mobile electrophile along a linear path of nitrogen nucleophiles [21] , [22] . The design of this system as well as that described below was inspired in part by the pioneering use of reversible Michael reactions for developing molecular yardsticks [23] , [24] . Recent success with the low-molecular walkers has demonstrated the potential to control the direction of transport by switches of pH and ultraviolet irradiation [25] , [26] . The inherent gain in transport efficiency for these examples over alternatives relying on Brownian diffusion [21] , [22] is not without consequence. Cycling between conditions or infusing energy may be tolerated in many applications but would not be feasible for most biological applications. For these, Brownian diffusion may remain optimum and highly satisfactory as evident from the success of DNA repair. Detection of nucleobase damage is a formidable task yet solved by nature using diffusional rather than directional scanning [27] , [28] , [29] . Whether directional or diffusional, transport based on covalent exchange still lacks a readily accessible and easily manipulated molecular surface to guide reaction. As described below, DNA is shown to provide a convenient surface for processive and bipedal diffusion of a dynamic crosslink in addition to its already well-characterized use in transport based on non-covalent exchange. DNA offers all of the benefits of easy assembly and creates defined surfaces containing nucleophilic footholds that are held more rigidly than those currently available with a linear aliphatic oligomer [11] , [22] , [30] . The use of DNA was initially suggested by the dynamics of its alkylation and crosslinking with a series of quinone methide (QM) derivatives [31] , [32] , [33] . QMs represent a readily available class of electrophiles capable of both capture and release of various nucleophiles [34] . These species are typically formed only transiently, and yet have found utility in the synthesis of natural products [35] , [36] , polymers [37] and cytotoxic agents [38] , as well as in functionalization of molecular surfaces [39] . QM formation and regeneration are exquisitely sensitive to electronic effects as evident from the five orders of magnitude separating rate constants for QMs differing by a single substituent [31] , [40] . Although the reversibility of QM reaction may complicate detection of their adducts formed by xenobiotic metabolism of certain drugs and food additives [41] , [42] , [43] , the reversibility has allowed for the construction of target-inducible and site-selective alkylating agents [44] , [45] , [46] . Prior model studies indicated that the strongest nucleophiles of DNA (G N7, A N1 and C N3) are alkylated by QMs most readily but their resulting adducts dissipate over time as the weakly nucleophilic nitrogens (G N 2 and A N 6 ) and water began to trap the regenerated QM irreversibly [43] , [47] . Here we tune the reversibility of QM formation by modulating the electronic nature of this intermediate. Thus, an initial failure to sustain migration of crosslinking in DNA is rectified by addition of an electron-donating group. The resulting QM is observed to walk along duplex DNA by the characteristic piperidine lability created from alkylation at the G N7 nucleophiles located in the major groove. Conjugation of the QM to acridine is necessary for efficient delivery of the initial crosslink, but this intercalator can also affect later migration by its preferential association at a nick in the phosphodiester backbone of duplex DNA. An alternative extrahelical bulge is sufficient to block crosslinking from achieving its thermodynamic distribution. Eventually, reversible crosslinking may be used to befuddle DNA repair and its response to noncanonical structures as a potential strategy for cancer chemotherapy. Tuning the binding and reversibility of DNA crosslinkers Most relevant to the current study was the design of bisfunctional precursors capable of generating two interrelated QM intermediates (bisQM) in series. These derivatives act as a potent crosslinker of DNA with an enviable ratio of crosslinking to monoalkylation [32] , [48] , [49] , [50] . The reversible nature of reaction additionally prolongs the effective lifetime of the electrophile many-fold and can maintain interstrand crosslinking while still permitting strand exchange ( Fig. 1 ). [51] , [52] This later feat suggests that the bisQM sequentially releases and recaptures the DNA in a manner that should support its covalent migration along the nucleophilic sites of DNA through a bipedal mechanism ( Fig. 2 ). 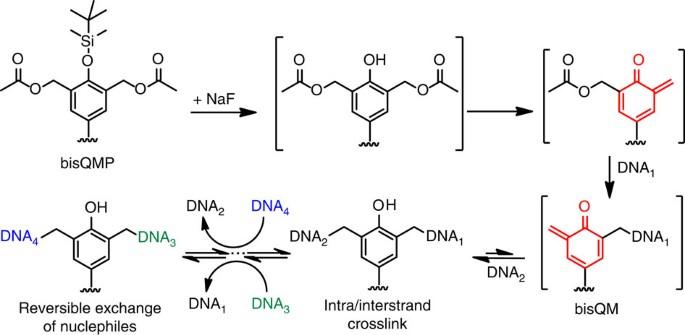Figure 1: Initial QM generation and subsequent exchange with DNA. QM formation (bisQM) is initiated by deprotection of a bisquinone methide precursor (bisQMP). Adducts formed by reaction with strong nucleophiles of DNA (dG N7, dA N1 and dC N3) regenerate the transient intermediate for iterative exchange of nucleophiles47,51. Other nucleophiles (for example, dG N2, dA N6, ROH) react weakly and irreversibly with equivalent QMs and T remains inert to these QMs. Figure 1: Initial QM generation and subsequent exchange with DNA. QM formation (bisQM) is initiated by deprotection of a bisquinone methide precursor (bisQMP). Adducts formed by reaction with strong nucleophiles of DNA (dG N7, dA N1 and dC N3) regenerate the transient intermediate for iterative exchange of nucleophiles [47] , [51] . Other nucleophiles (for example, dG N 2 , dA N 6 , ROH) react weakly and irreversibly with equivalent QMs and T remains inert to these QMs. 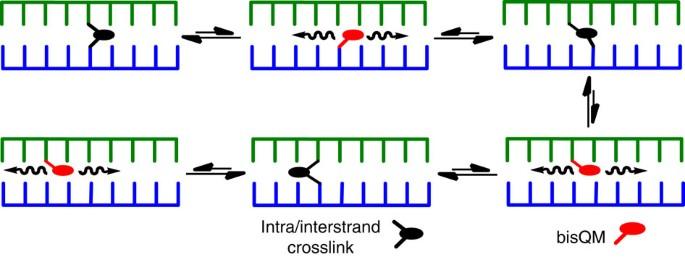Figure 2: Mobility of DNA crosslinking. Capture and release of a bisQM intermediate allows for bipedal-like walking within duplex DNA. Full size image Figure 2: Mobility of DNA crosslinking. Capture and release of a bisQM intermediate allows for bipedal-like walking within duplex DNA. Full size image The oligonucleotide system used previously to monitor strand exchange by dynamic crosslinking of bisQM [52] serves equally well as a prototype for testing the electrophile’s ability to walk autonomously along a track of nucleophiles. The first challenge for this involved delivery of the mobile bisQM to a limited region of DNA, yet retain contiguous and untreated areas for subsequent migration. This was accomplished by treating one oligonucleotide donor strand with bisQM to form intrastrand crosslinks that subsequently isomerize to interstrand crosslinks after hybridization to a complementary target sequence [52] . This process avoids the possibility of forming alkylation products in a single-stranded region since the target strand is never exposed to the electrophile directly (see below). Subsequent addition of a third strand of DNA extends the duplex structure and establishes a new region of track for observing migration of the covalent adduct. A bisQM was prepared as before by fluoride-dependent deprotection of a silylated bisQM precursor that was conjugated to acridine (bisQMP1, 1 ; Fig. 3 ). Although this species had previously supported exchangeable crosslinking [52] , it did not appear to migrate from its original positions to a nascent duplex from preliminary analysis extending over 7 days (see below). This period was initially thought sufficient to detect transport since duplexes containing an interstrand crosslink required no more than 1–2 days for complete strand exchange [52] . In retrospect, this benchmark may not have been appropriate for detecting autonomous walking since the exchange studies relied on successive additions of oligonucleotides to form increasingly stable duplexes. In contrast, crosslink migration was examined along a single DNA duplex without intervention and driven by only the energy associated with diffusion towards its equilibrium distribution. Intrahelical migration may then exhibit a greater dependence on the bisQM structure than previously expressed by the related exchange studies. 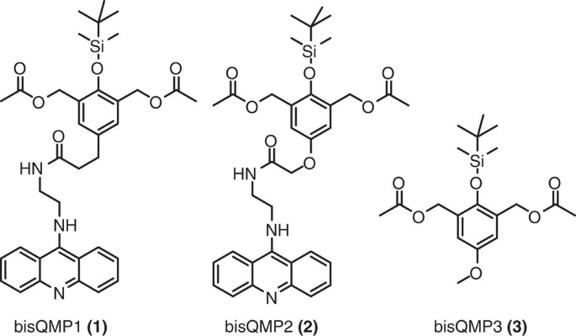Figure 3: bisQuinone methide precursors. Reagents used for dynamic crosslinking of DNA. Figure 3: bisQuinone methide precursors. Reagents used for dynamic crosslinking of DNA. Full size image Two analogues of the original bisQMP1 ( 1 ) were generated to address possible limitations in covalent exchange and repositioning necessary for bipedal walking. First, strand release from the covalent crosslink could have been too slow and the lifetime of the resulting bisQM intermediate could have been too short to allow for its reorientation along the track to reach a new foothold. The kinetics of covalent exchange were therefore enhanced by increasing the electron-donating nature of the linker from a benzylic methylene group in bisQMP1 ( 1 ) to an ether oxygen in bisQMP2 ( 2 ) ( Fig. 3 ) [31] . Second, the time required for reorientation could have been exacerbated by slow exchange of acridine between sites of intercalation. Acridine was originally attached to the bisQM to increase its local concentration proximal to duplex DNA and consequently minimize the molar equivalents required for efficient crosslinking [32] , [53] . The role of intercalation was similarly examined with the help of an additional derivative lacking the acridine component (bisQMP3, 3 ). These target compounds were readily synthesized in analogy to the parent compound bisQMP1 ( 1 ) ( Fig. 4 ). 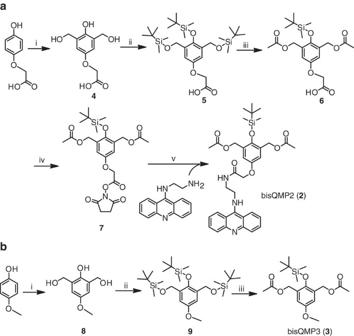Figure 4: Synthesis of bisquinone methide precursors. (a) Reagents and conditions: (i) CH2O, CaO, 5 days, 67%. (ii)tert-butyldimethylsilyl chloride, imidazole, 35 h, DMF, 75%. (iii) Ac2O, FeCl3, 1 h, 85%. (iv)N-hydroxysuccinamide, 1-ethyl-3-(3-dimethylaminopropyl)carbodiimide (EDC), CH2Cl2, 18 h, 56%. (v) Et3N, 1.5 h, 42%. (b) Reagents and conditions: (i) CH2O, CaO, 5 days, 67%. (ii)tert-butyldimethylsilyl chloride, imidazole, 16 h, DMF, 60%. (iii) Ac2O, FeCl3, 2 h, 66%. Figure 4: Synthesis of bisquinone methide precursors. ( a ) Reagents and conditions: (i) CH 2 O, CaO, 5 days, 67%. (ii) tert -butyldimethylsilyl chloride, imidazole, 35 h, DMF, 75%. (iii) Ac 2 O, FeCl 3 , 1 h, 85%. (iv) N -hydroxysuccinamide, 1-ethyl-3-(3-dimethylaminopropyl)carbodiimide (EDC), CH 2 Cl 2 , 18 h, 56%. (v) Et 3 N, 1.5 h, 42%. ( b ) Reagents and conditions: (i) CH 2 O, CaO, 5 days, 67%. (ii) tert -butyldimethylsilyl chloride, imidazole, 16 h, DMF, 60%. (iii) Ac 2 O, FeCl 3 , 2 h, 66%. Full size image Efficiency of DNA crosslinking by the modified QMs The potential success of the new derivatives to sustain transport was initially evaluated by the yields and kinetics of their DNA crosslinking. The electron-rich derivative bisQMP2 ( 2 ) demonstrated the desired increase in potency above that of the original bisQMP1 ( 1 ). Within 5 h, bisQMP2 ( 2 ) (12 μM) produced an average of 60% crosslinking in contrast to bisQMP1 ( 1 ) that formed an average of only 18% crosslinking under equivalent conditions ( Supplementary Fig. 1 ). Ultimately, bisQMP2 ( 2 ) succeeded in crosslinking greater than 95% of the duplex DNA after 18 h. For perspective, the highly regarded reagents cisplatin and mitomycin C typically generate DNA crosslinking with yields of no greater 10% [54] , [55] , [56] . The inductive effect of the ether oxygen did not circumvent the need for the acridine appendage. The bisQMP3 ( 3 ) formed crosslinking with yields similar to that of bisQMP1 ( 1 ) but required a 400-fold greater concentration (4.8 mM) for this result. Still, this yield is significantly greater (threefold) than that for the parent of bisQMP3 ( 3 ) lacking the p -methoxy group [53] . The further enhancement offered by the attached acridine likely derives from its ability to localize the bisQM to the DNA and perhaps even direct it to the major groove near the accessible G N7. Efficiency of QM exchange The ability of the electron-rich substituent to promote DNA crosslinking by tandem QM formation was necessary but not sufficient for supporting migration along a duplex. The bisQM also needed to sustain repetitive regeneration from and recapture by DNA. The influence of the oxygen substitution on these processes was demonstrated through an intra- to interstrand crosslink isomerization first used to identify the dynamics of bisQM1 crosslinking [51] , [52] . The electrophilic intermediates were initially captured by pretreatment with OD1 for 24 h, a period sufficient for complete consumption of the bisQMPs through reversible alkylation of DNA and irreversible quenching by water ( Fig. 5 ) [51] . Only the fraction of bisQMP captured by OD1 retains the dynamics for subsequent transfer of a QM linkage to the complementary OD2. Isomerization of crosslinks from intra- to interstrand positions was detected by time-dependent accumulation of a low-mobility species on denaturing polyacrylamide gel electrophoresis ( Fig. 5 ). Equivalent crosslinking is not observed if donor and acceptor DNA strands lack complementarity and, to date, crosslinking has not been capable of hopping between unrelated DNA duplexes [51] , [52] . In this assay, the electron-rich bisQM2 appears to accelerate transfer in the first 4 h of reaction by minimizing the lag observed for the original bisQM1. Comparable interstrand crosslinking by bisQM3 lacking the intercalator was very inefficient and may have been suppressed by adventitious reactions caused by the initial presence of a large excess of bisQMP3. 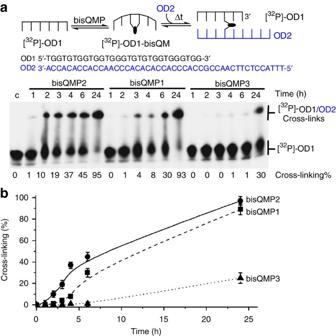Figure 5: QM transfer depends on the dynamics of benzylic substitution. (a) Intrastrand crosslinks of OD1 isomerize to interstrand crosslinks after addition of complementary DNA (OD2, 3.3 mM) to [32P]-OD1 (50 nCi, 3.0 μM) in MES (pH 7.0, 10 mM) and 20% acetonitrile that had been pretreated alternatively with bisQMP2 (2) (12 μM), bisQMP1 (1) (12 μM) or bisQMP3 (3) (4.8 mM) in the presence of NaF (50 mM) for 24 h. An equivalent mixture lacking NaF was analysed in lane c. Crosslinked products were detected by their characteristic low mobility during denaturing polyacrylamide gel electrophoresis (20%). (b), Formation of interstrand crosslinks was quantified by phosphoimagery and calculated relative to total signal. Error bars represent the range of two independent experiments and the lines between data are added only as a visual aid to highlight the trends in reactivity. Figure 5: QM transfer depends on the dynamics of benzylic substitution. ( a ) Intrastrand crosslinks of OD1 isomerize to interstrand crosslinks after addition of complementary DNA (OD2, 3.3 mM) to [ 32 P]-OD1 (50 nCi, 3.0 μM) in MES (pH 7.0, 10 mM) and 20% acetonitrile that had been pretreated alternatively with bisQMP2 ( 2 ) (12 μM), bisQMP1 ( 1 ) (12 μM) or bisQMP3 ( 3 ) (4.8 mM) in the presence of NaF (50 mM) for 24 h. An equivalent mixture lacking NaF was analysed in lane c. Crosslinked products were detected by their characteristic low mobility during denaturing polyacrylamide gel electrophoresis (20%). ( b ), Formation of interstrand crosslinks was quantified by phosphoimagery and calculated relative to total signal. Error bars represent the range of two independent experiments and the lines between data are added only as a visual aid to highlight the trends in reactivity. Full size image The effects of the electron-rich substituent on bisQM were even more apparent when the dynamics of its regeneration within duplex DNA was monitored by its ability to allow strand exchange and yet reestablish interstrand crosslinking. To begin, an equimolar concentration of a labelled strand OD3 was added to the crosslinked duplex OD1/OD2 formed above. Time-dependent incorporation of OD3 into the crosslink was promoted threefold for the bisQM2 intermediate ( t ½ ~44 h) relative to the original parent bisQM1 ( t ½ ~150 h, Fig. 6 ). This is most evident after 24 h when 30% of OD3 is associated with the low-mobility product established by bisQM2 crosslinking in comparison with a yield of 10% for the equivalent product established by bisQM1. Exchange reaches an equilibrium after ~36 h for bisQM2 crosslinking, whereas an approach to equilibrium for the bisQM1 system remains far from complete after 48 h. The maximum yield of either exchange is only ~50% since each complementary strand has an equal probability of retaining the bisQM intermediate after strand displacement. The fraction associated with OD2 subsequently forms interstrand crosslinks with OD3. Conversely, the fraction associated with OD1 forms intrastrand crosslinks since OD1 is not competitive with OD3 for rehybridization to OD2. 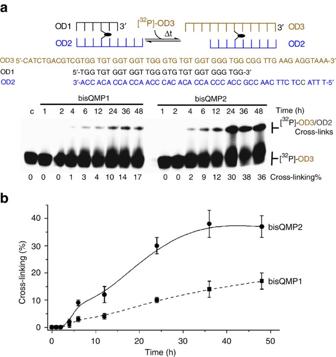Figure 6: An electron-rich bisQM facilitates strand exchange with DNA. (a) OD3/OD2 crosslinks were formed under ambient conditions by exchange of equimolar32P-OD3 (3.0 μM, 50 nCi) into crosslinked OD1/OD2 (3 μM). Initial crosslinking was formed indirectly by standard treatment of OD1 (3.0 μM) with the bisQMP (12 μM) and NaF (50 mM) in MES (10 mM, pH 7) and 20% acetonitrile for 24 h before OD2 (3.3 μM) was added and incubation continued for an additional 24 h. Lane c lacked addition of NaF. Crosslinked products were detected by their characteristic low mobility during denaturing polyacrylamide gel electrophoresis (20%). (b) Rates of strand exchange were measured by phosphoimagery and calculated relative to total signal. Error bars represent the range of two independent experiments and the lines are added only as a visual aid to highlight the trends in reactivity. Figure 6: An electron-rich bisQM facilitates strand exchange with DNA. ( a ) OD3/OD2 crosslinks were formed under ambient conditions by exchange of equimolar 32 P-OD3 (3.0 μM, 50 nCi) into crosslinked OD1/OD2 (3 μM). Initial crosslinking was formed indirectly by standard treatment of OD1 (3.0 μM) with the bisQMP (12 μM) and NaF (50 mM) in MES (10 mM, pH 7) and 20% acetonitrile for 24 h before OD2 (3.3 μM) was added and incubation continued for an additional 24 h. Lane c lacked addition of NaF. Crosslinked products were detected by their characteristic low mobility during denaturing polyacrylamide gel electrophoresis (20%). ( b ) Rates of strand exchange were measured by phosphoimagery and calculated relative to total signal. Error bars represent the range of two independent experiments and the lines are added only as a visual aid to highlight the trends in reactivity. Full size image Bipedal migration along DNA containing a backbone nick The successive rather than concurrent formation of the two QM intermediates generated by bisQMPs enforces their stepwise transfer and avoids full dissociation from DNA. This feature similarly aids delivery of interstrand crosslinks to a defined region of duplex DNA (OD1/OD2, Fig. 5 ) through transfer from an intrastrand intermediate. This same process provided a convenient method for establishing initial positions of crosslinking before introducing an extended track for walking. Accordingly, crosslinks were generated first by capturing bisQMs with OD4 to form intrastrand crosslinks ( Supplementary Fig. 2 ) and then second by adding OD2 to form interstrand crosslinks between the complementary regions of OD2 and OD4. This strategy avoided direct exposure of OD2 to the bisQMPs and prevented spontaneous reaction in the single-stranded region of OD2 extending beyond OD4. The carrier OD4 was used instead of the original OD1 in this and later experiments simply to direct subsequent migration towards the 5′ terminus of the nascent duplex region for ease in detection after piperidine induced fragmentation as illustrated below. Addition of OD5 effectively extends the initial duplex formed by OD4/OD2 and provides a new region for the mobile bisQM crosslink to wander ( Fig. 7 ). Net migration of the crosslink to the OD5/OD2 helix was first identified by the low-mobility and high-molecular weight crosslink product after denaturing gel electrophoresis ( Supplementary Fig. 3 ). Such a species was not observed in the alternative presence of the parent bisQM1 or its electron-rich derivative lacking acridine (bisQM3). These electrophiles were evidently not sufficiently mobile to gain access to OD5. Only crosslinks formed by bisQM2 were able to migrate from the helical region of OD2/OD4 to the adjacent helical region of OD2/OD5. 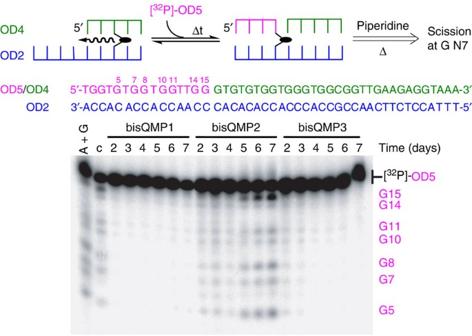Figure 7: Crosslink migration is only evident for the most electron-rich bisQM2. Initial crosslinking between OD2 and OD4 was generated by initial treatement of OD4 (3.0 μM) with bisQMP2 (2) (12 μM) and NaF (50 mM) in MES (10 mM, pH 7) and 20% acetonitrile under ambient conditions for 24 h in analogy to that described for OD1. OD2 (3.3 μM) was then added and incubation was continued for another 24 h before 5′-[32P]-OD5 (50 nCi, 3.0 μM) was added. Lane c represents direct reaction between bisQMP2 (2) (12 μM) and a preannealed duplex of [32P]-OD5+OD4/OD2 in MES (pH 7.0, 10 mM), NaF (50 mM) and 20% acetonitrile for 6 h. All samples were treated with hot piperidine, separated by denaturing gel electrophoresis (20%) and quantified by phosphoimagery. Figure 7: Crosslink migration is only evident for the most electron-rich bisQM2. Initial crosslinking between OD2 and OD4 was generated by initial treatement of OD4 (3.0 μM) with bisQMP2 ( 2 ) (12 μM) and NaF (50 mM) in MES (10 mM, pH 7) and 20% acetonitrile under ambient conditions for 24 h in analogy to that described for OD1. OD2 (3.3 μM) was then added and incubation was continued for another 24 h before 5′-[ 32 P]-OD5 (50 nCi, 3.0 μM) was added. Lane c represents direct reaction between bisQMP2 (2) (12 μM) and a preannealed duplex of [ 32 P]-OD5+OD4/OD2 in MES (pH 7.0, 10 mM), NaF (50 mM) and 20% acetonitrile for 6 h. All samples were treated with hot piperidine, separated by denaturing gel electrophoresis (20%) and quantified by phosphoimagery. Full size image In a complementary analysis, the distribution of alkylation within OD5 at G N7 was monitored over time by its diagnostic strand scission induced by subsequent piperidine treatment. Reversible alkylation of G N7 had previously dominated the reaction of bisQMP1 ( 1 ) with duplex DNA and dynamic reaction at the C N3 and A N1 were also detected with related QM intermediates [32] , [43] , [47] . All of these nucleophiles likely participate in crosslinking, particularly since OD2 contains only a single G and this G is far from the region that could crosslink with OD5. In contrast, the abundance of Gs in OD5 helped to trace the migration of bisQM along its track of nucleophiles. OD5 was not sensitive to piperidine treatment when first added to the crosslinked OD2/OD4 as expected from its initial lack of G N7 modification ( Fig. 7 ). Also, no piperidine sensitivity developed for OD5 after extended incubation with OD2/OD4 containing crosslinks formed by bisQM1 or bisQM3. This is consistent with the lack of crosslink migration identified for these electrophiles ( Supplementary Fig. 3 ). Equivalent crosslinks formed by bisQM2 were sufficiently mobile to walk onto OD5 and induce increasing levels of piperidine-dependent scission during incubation ( Figs 7 and 8 ). After 7 days, the array of fragments was qualitatively equivalent to the thermodynamic distribution formed by treating a preannealed complex of OD2, OD4 and OD5 with bisQMP2 ( 2 ) directly ( Figs 7 and 8 , lane c). Although the approach to equilibrium may seem slow, no chemical intervention or addition of energy was needed for migration of bisQM2 along the extent of OD5+OD4/OD2. In addition, this process represents a culmination of many covalent exchanges. For example, bipedal walking from the 5′-G of OD4 to G5 of OD5 requires a minimum of 14 steps if transient bonds to each intervening G on OD5 and a corresponding set of nucleobases on OD2 are involved. For perspective, 2 days were necessary for an α-methylene-4-nitrostyrene to traverse along just two nucleophilic footholds in a diethylenetriamine track [22] . 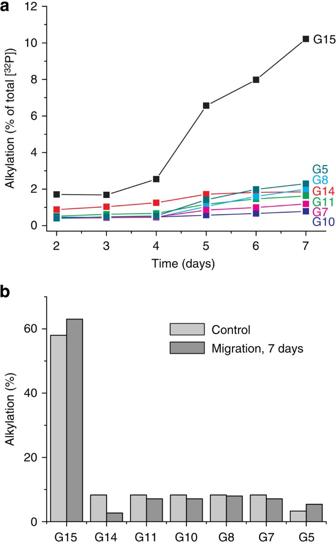Figure 8: Crosslink migration within a nick-containing helix. (a) The time-dependent distribution of alkylation at G N7 after addition of 5′-[32P]-OD5 to the crosslinked OD4/OD2 was quantified using the electrophoretic profile ofFig. 7that was generated by bisQMP2 (2). (b) The fractional distribution of strand scission from a control reaction of preassembled 5′-[32P]-OD5 +OD4/OD2 with bisQMP2 (2) (Fig. 7, lane c) is compared with that formed after a 7-day migration of equivalent crosslinks from OD4/OD2 to the added 5′-[32P]-OD5 (Fig. 7). Figure 8: Crosslink migration within a nick-containing helix. ( a ) The time-dependent distribution of alkylation at G N7 after addition of 5′-[ 32 P]-OD5 to the crosslinked OD4/OD2 was quantified using the electrophoretic profile of Fig. 7 that was generated by bisQMP2 ( 2 ). ( b ) The fractional distribution of strand scission from a control reaction of preassembled 5′-[ 32 P]-OD5 +OD4/OD2 with bisQMP2 ( 2 ) ( Fig. 7 , lane c) is compared with that formed after a 7-day migration of equivalent crosslinks from OD4/OD2 to the added 5′-[ 32 P]-OD5 ( Fig. 7 ). Full size image The nucleophilic footholds offered by DNA are very efficient at capturing the QM intermediate due to their high effective molarity along the walk from the helical region of OD4 to that of OD5. This process was not detectably quenched by irreversible trapping with β-mercaptoethanol when added in more than 300-fold excess over the DNA duplex ( Supplementary Fig. 4 ). This lack of susceptibility to low-molecular weight nucleophiles is consistent with that observed during previous crosslink delivery and exchange studies using QM intermediates associated with DNA but not necessarily attached to an intercalator [44] , [51] . In the absence of DNA, these intermediates are quenched very rapidly by competing nucleophiles [47] . The G15 of OD5 appears to be the primary target of alkylation by bisQM2 regardless of whether it reacted directly or after covalent migration from a distant site ( Fig. 7 ). Such localization is consistent with the preferred association of the acridine appendage near a nick in the phosphodiester backbone such as that made by the junction of OD4 and OD5. This site is most easily unwound to accommodate the intercalator and represents just one of many noncanonical structures of DNA that preferentially bind intercalators. Other examples include abasic sites, mismatched base pairs and regions containing extrahelical bases [57] , [58] , [59] , [60] . Thus, there is a potential for a mobile crosslinker to scan over DNA for damage by walking along canonical structures and ultimately accumulating at aberrant sites that offer the most favourable thermodynamics for alkylation and intercalation. Of course, acridine could also be substituted in the future with a variety of other ligands for sensing a range of anomalies within duplex DNA. Bipedal migration along a continuous region of canonical DNA To confirm the migratory ability of bisQM2 through a canonical duplex structure, OD6, the full complement of OD2, was substituted for OD5 in the system above. In this strategy, OD4 effectively acts as a shuttle by delivering bisQM2 to a limited region in OD2 and then departing after strand exchange with OD6 (ref. 52 ). The expected localization of bisQM2 within the original boundaries defined by OD4 was confirmed by the initial profile of fragments induced by piperidine. These were initially limited to the region from G16 to the 3′ terminus of OD6 ( Fig. 9 ). After 2 days, scission at G14 and G15 became apparent. After 7 days, scission extended to G5. This time-dependent progression of piperidine sensitivity best illustrates the linear diffusion and stepwise progress of bisQM2. An equivalent evolution of products would not have formed if the bisQM2 had fully dissociated before returning to the duplex or if it had been exchanged through some type of assembly between multiple duplexes. Finally, reaction progress of OD6 was also not sustained by any lingering source of bisQM2 beyond that initially delivered by OD4 since the total level of alkylation-induced scission remained constant over the 7-day incubation ( Fig. 9b ). 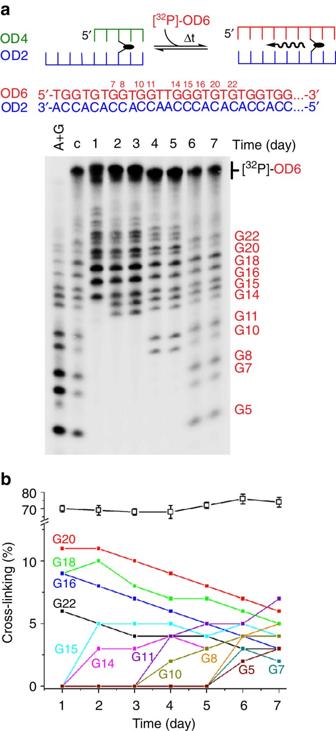Figure 9: Dynamic crosslinking migrates freely within a canonical duplex of DNA. (a) Initial crosslinking between OD2 and OD4 was generated by the treatment of OD4 (3.0 μM) with bisQMP2 (2) (12 μM) in MES (pH 7.0, 10 mM), NaF (50 mM) and 20% acetonitrile for 24 h before addition of OD2 (3.3 μM) and incubation for an additional 24 h. A stoichiometric concentration of [32P]-OD6 (50 nCi, 3.0 μM) was then added for exchange with OD4. Lane c represents direct reaction between bisQMP2 (2) (12 μM) and a preannealed duplex of [32P]-OD6/OD2 in MES (pH 7.0, 10 mM), NaF (50 mM) and 20% acetonitrile for 5 h. All samples were treated with hot piperdine, separated by denaturing gel electrophoresis (20%) and quantified by phosphoimagery. (b) Strand scission induced by crosslinking was determined over time relative to the total signal. Scission at individual sites and collectively (□) was calculated relative to the total DNA signal. Error bars represent the s.d. of three independent experiments. Errors associated with scission at individual sites are less than 10% of their values and not shown to maintain clarity. Figure 9: Dynamic crosslinking migrates freely within a canonical duplex of DNA. ( a ) Initial crosslinking between OD2 and OD4 was generated by the treatment of OD4 (3.0 μM) with bisQMP2 ( 2 ) (12 μM) in MES (pH 7.0, 10 mM), NaF (50 mM) and 20% acetonitrile for 24 h before addition of OD2 (3.3 μM) and incubation for an additional 24 h. A stoichiometric concentration of [ 32 P]-OD6 (50 nCi, 3.0 μM) was then added for exchange with OD4. Lane c represents direct reaction between bisQMP2 ( 2 ) (12 μM) and a preannealed duplex of [ 32 P]-OD6/OD2 in MES (pH 7.0, 10 mM), NaF (50 mM) and 20% acetonitrile for 5 h. All samples were treated with hot piperdine, separated by denaturing gel electrophoresis (20%) and quantified by phosphoimagery. ( b ) Strand scission induced by crosslinking was determined over time relative to the total signal. Scission at individual sites and collectively (□) was calculated relative to the total DNA signal. Error bars represent the s.d. of three independent experiments. Errors associated with scission at individual sites are less than 10% of their values and not shown to maintain clarity. Full size image Without intervention, the dynamic crosslinks diffused to all regions of the DNA duplex yet still remained attached through covalent bonding. This was made possible by the release and recapture of the QM intermediate formed interchangeably but not simultaneously at either benzylic position of the crosslinker ( Figs 1 and 2 ). No single site along the canonical duplex accumulated a major fraction of crosslinking since none offered a significant advantage for intercalation. Walking along duplex DNA towards an extrahelical bulge The potential barriers for migration of bisQM2 across DNA were pushed beyond a canonical or nicked duplex to include an analogue containing a bulge structure formed by two extrahelical Ts. Ts were chosen for their lack of reaction with the parent QM [61] and inserted into the sequence of OD6 resulting in a new strand OD7. This new strand was then used to displace OD4 from its crosslinked duplex with OD2. The product of strand exchange was equivalent to that formed by OD2/OD6 above except for the presence of the unpaired Ts between sets of Gs as illustrated in Fig. 10 . Again, the bisQM2 was initially transferred to the N7 of Gs in the 3′-region of OD7 as expected ( Fig. 10 ). Migration of bisQM2 from this region was then evident as piperidine-labile sites spread to adjacent Gs (G16, G17) and later to more distal Gs (G12, G13). Similar to previous studies, the level of strand scission remained constant throughout the entire 7-day incubation, and thus bisQM2 migrated to new sites without a net gain or loss of covalent attachment to G N7 ( Fig. 10b ). However, the obstacle created by the extrahelical Ts was sufficient to block the stride of bisQM2 required to reach G8 from G12. This represents a kinetic hurdle since the thermodynamic profile formed by direct reaction of bisQMP2 ( 2 ) and preannealed OD2/OD7 was dominated by reaction at G8 ( Fig. 10 , lane c). The inability of bisQM2 to attain the thermodynamic profile from bipedal walking also confirmed that bisQM2 acted processively and never completely dissociated from its DNA track. Otherwise, reaction would have freely accumulated at the preferred site of G8. 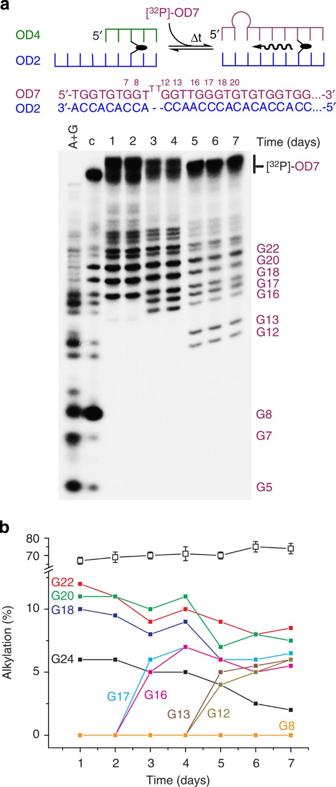Figure 10: A noncanonical structure impedes the migration of dynamic crosslinking in DNA. (a), All conditions and protocols were analogous to those described inFig. 9except that [32P]-OD7 was used in place of [32P]-OD6. Initial crosslinking between OD2 and OD4 was generated by the treatment of OD4 (3.0 μM) with bisQMP2 (2) (12 μM) in MES (pH 7.0, 10 mM), NaF (50 mM) and 20% acetonitrile for 24 h before addition of OD2 (3.3 μM) and incubation for an additional 24 h. A stoichiometric concentration of [32P]-OD7 (50 nCi, 3.0 μM) was then added for exchange with OD4. (b) Strand scission induced by crosslinking was determined over time relative to the total signal. Scission at individual sites and collectively (□) was calculated relative to the total DNA signal. Error bars represent the s.d. of three independent experiments. Errors associated with scission at individual sites are less than 10% of their values and are not shown to maintain clarity. Figure 10: A noncanonical structure impedes the migration of dynamic crosslinking in DNA. ( a ), All conditions and protocols were analogous to those described in Fig. 9 except that [ 32 P]-OD7 was used in place of [ 32 P]-OD6. Initial crosslinking between OD2 and OD4 was generated by the treatment of OD4 (3.0 μM) with bisQMP2 ( 2 ) (12 μM) in MES (pH 7.0, 10 mM), NaF (50 mM) and 20% acetonitrile for 24 h before addition of OD2 (3.3 μM) and incubation for an additional 24 h. A stoichiometric concentration of [ 32 P]-OD7 (50 nCi, 3.0 μM) was then added for exchange with OD4. ( b ) Strand scission induced by crosslinking was determined over time relative to the total signal. Scission at individual sites and collectively (□) was calculated relative to the total DNA signal. Error bars represent the s.d. of three independent experiments. Errors associated with scission at individual sites are less than 10% of their values and are not shown to maintain clarity. Full size image The effect of the extrahelical bulge within duplex DNA provides a stark contrast to that induced by the more subtle nick in the phosphodiester backbone. The TT bulge dramatically altered the thermodynamic array of crosslink products and established a structural barrier preventing migration to adjacent footholds provided by the surrounding canonical DNA ( Fig. 10 ). In contrast, the nick did not prevent bisQM2 from traversing the entire length of the DNA duplex although it still affected the thermodynamic array of products ( Fig. 7 ). The behaviour of this molecular walker is likely a function of the binding specificity of the acridine, the stability of the intermediate electrophile and the distance between sites for nucleophilic capture. Each of these may be adapted in the future to respond to different structures and molecular signals created by tracks of nucleic acids. In addition, the kinetics of nucleophilic exchange can be adjusted by substituents attached to the QM as illustrated in this work with bisQM1 and bisQM2. Ligand exchange by transition metals provides an alternative basis for bipedal diffusion along DNA but few examples have yet been published. To date, Pt(II) migration has only been observed over a single bipedal transfer [54] , [62] , [63] . A related system utilizing Pd(II) with a track of pyridine ligands alternatively required addition of heat and a pH change to drive bipedal walking [64] . Neither metal will likely support exchange processes over the range of kinetic regimes available for QM intermediates under neutral aqueous conditions. QM reaction with DNA once again demonstrates great versatility. The strong nucleophiles of DNA successfully compete for addition to QM yet also act as strong leaving groups for regeneration of QM in a dynamic process that persists over many days [51] , [52] . The newly observed migration of a bisQM along duplex DNA illustrates that this dynamic process can extend over distances of at least 10 base pairs ( Fig. 9 ). Analogous to electron transport in DNA [65] , [66] , migration of the QM electrophile is sensitive to nucleotide sequence and structure as well. Mutually exclusive formation of each QM enforces a bipedal walk along the track of nucleophiles presented by the DNA. This action requires no chemical or physical intervention nor does it consume the track during migration towards its equilibrium distribution of crosslinking. The ability of DNA to support bipedal walking through dynamic covalent chemistry opens many opportunities for fundamental exploration and application development since tracks of nucleophiles can be easily generated into diverse shapes and dimensions by self-assembly. General methods and materials NMR spectra were recorded on a Bruker AM400, AM500 or AM600 spectrometer and referenced to residual protons in the deuterated solvents. Chemical shifts ( δ ) and coupling constants ( J ) are reported in parts per million (p.p.m.) and Hertz (Hz), respectively. High-resolution mass spectra were determined by electrospray ionization with Hewlett-Packard 5980A and VG 7070E mass spectrometers. Melting points (uncorrected) were measured with a Thomas-Hoover Unimelt apparatus. Organic reagents and starting materials were purchased from Sigma-Aldrich and used without further purification. Solvents, buffers and salts were purchased from Fisher Scientific and Sigma-Aldrich. Silica gel plates (230–400 mesh, 20 × 20 cm) for preparative thin layer chromatography (TLC) were purchased from Fisher Scientific. Oligodeoxyribonucleotides were purchased from IDT and labelled at their 5′ terminus with 5′-[ γ - 32 P]-ATP and T4 polynucleotide kinase as directed by the enzyme supplier (New England Biolabs). All aqueous solutions used water purified to a resistivity of greater than 17.8 MΩ. DNA concentrations were calculated from their absorption at 260 nm and their ε 260 values provided by the vender. bisQMP1 ( 1 ) was synthesized by Dr Huan Wang as described previously [51] . Synthesis of 4 Calcium oxide 0.20 g, 3.6 mmol) was added to a mixture of 2-(4-hydroxyphenoxy)acetic acid (0.72 g, 4.3 mmol) and aqueous formaldehyde (37%, 2 ml) in a plastic tube [67] . The reaction was shaken at room temperature in the dark for 5 days, cooled (5 °C), neutralized with 2 M HCl (8 ml) and kept in an ice bath for 30 min. The resulting yellow precipitate was filtered to yield 4 (0.63 g, 67%). 1 H NMR (400 MHz, MeOD) δ 6.79 (s, 2H), 4.66 (s, 4H), 4.58 (s, 2H). 13 C NMR (126 MHz, MeOD) δ 172.71, 152.61, 148.44, 129.68, 113.99, 66.41, 61.51. HRMS m/z calculated for C 10 H 12 O 6 228.0365, found 227.0334 ([M−H] + ); melting point, 87–88 °C. Synthesis of 5 Imidazole (2.40 g, 35.3 mmol) was added to a solution of tert -butyldimethylsilyl chloride (TBDMSCl, 3.60 g, 24.0 mmol) and 4 (0.71 g, 3.1 mmol) in 6 ml of DMF. The reaction mixture was stirred at room temperature for 35 h, diluted with brine (50 ml), and extracted with ether (3 × 50 ml). The organic phases were combined, dried over MgSO 4 , and concentrated under reduced pressure. The residue was then dissolved in methanol (30 ml) treated with potassium carbonate (1.0 g). The resulting mixture was stirred for 2 h at ambient temperature, neutralized with 2 M HCl (20 ml), diluted with water (50 ml) and extracted with ether (3 × 50 ml). The organic phases are combined, washed with brine (50 ml), dried over MgSO 4 and concentrated under reduced pressure. The residue was purified by silica gel flash chromatography (1% AcOH in hexanes:ethyl acetate, 1:0–7:3) to yield 5 as a white solid (0.44 g, 75%). 1 H NMR (400 MHz, CDCl 3 ) δ 6.95 (s, 2H), 4.65–4.62 (s, 6H), 0.91 (s, 27H), 0.06 (s, 18H). 13 C NMR (126 MHz, CDCl 3 ) δ 146.32, 124.06, 114.39, 104.71, 83.75, 37.16, 32.48, −1.84, −9.38, −9.91, −28.02, −31.64, −33.46. HRMS m/z calculated for C 28 H 54 O 6 Si 3 570.3003, found 569.3063 ([M –H] + ); melting point, 135–137 °C. Synthesis of 6 Solid ferric chloride (40.5 mg, 0.250 mmol) was added to a solution of 5 (0.63 g, 1.1 mmol) in acetic anhydride (9 ml) at 0 °C under nitrogen. The reaction mixture was stirred for 1 h and then mixed with ether (50 ml). The combined organic phases were washed with water (2 × 50 ml) and saturated NaHCO 3 (3 × 50 ml, caution gas release), dried with MgSO 4 and concentrated under reduced pressure. The residue was separated by silica gel flash chromatography (hexane:ethyl acetate, 1:0–7:3) to yield 6 as a colourless oil (0.40 g, 85%). 1 H NMR (500 MHz, CDCl 3 ) δ 6.91(s, 2H), 5.07 (s, 4H), 4.76 (s, 2H), 2.10 (s, 6H), 1.02 (s, 9H), 0.18 (s, 6H). 13 C NMR (126 MHz, CDCl 3 ) δ 170.87, 164.32, 151.71, 145.89, 128.21, 115.60, 66.13, 62.12, 26.00, 22.07, 21.00, 0.77, −3.56. HRMS m/z calculated for C 20 H 30 O 8 Si 426.1675 found 425.1589 ([M–H] + ). Synthesis of 7 N -Hydroxysuccinimide (0.210 g, 1.83 mmol) was added to a solution of 6 (0.38 g, 0.89 mmol) in dry methylene chloride (10 ml). The solution was stirred in an ice bath under N 2 and 1-ethyl-3-(3-dimethylaminopropyl)carbodiimide (EDC, 0.35 g, 1.8 mmol) was added. The reaction was stirred for 18 h at room temperature and then brine (50 ml) was added as a quench. The mixture was extracted with ether (3 × 50 ml). The combined organic phase was then extracted with brine (50 ml) and dried over MgSO 4 and filtered. The filtrate was concentrated under low pressure and purified by preparative silica gel TLC (3:7 ethyl acetate in hexanes) to yield the desired activated ester of 7 (0.26 g, 56%) as a viscous yellow liquid. 1 H NMR (500 MHz, CDCl 3 ) δ 6.93 (s, 2H), 5.07 (s, 4H), 4.94 (s, 2H), 2.33 (s, 4H), 2.10 (s, 6H), 1.01 (s, 9H), 0.17 (s, 6H). 13 C NMR (126 MHz, CDCl 3 ) δ 171.06, 169.31, 165.78, 151.91, 146.22, 128.23, 116.11, 64.24, 61.76, 26.09, 25.77, 21.15, 17.77, −3.54. HRMS m/z calculated for C 24 H 33 NO 10 Si 523.1920, found 524.1889 ([M+H] + ). Synthesis of bisQMP2 ( 2 ) Triethylamine (1 ml) was added to a suspension of N -(9-acridinyl)-1,2-diaminoethane [32] (30.0 mg, 0.126 mmol) in acetonitrile (4 ml). Once all the material dissolved, the activated ester of 7 (0.07 g, 0.1 mmol) in acetonitrile (4 ml) was added dropwise over 1 min and the mixture was stirred for 1.5 h at room temperature. Acetic acid (3 ml) and water (40 ml) were then added and the mixture was extracted with methylene chloride (4 × 40 ml). The organic phase was separated and extracted with brine (3 × 50 ml), washed with sodium phosphate (500 mM pH 7.0, 30 ml), dried over MgSO 4 and filtered. The filtrate was concentrated under reduced pressure and separated by preparative scale TLC (CH 2 Cl 2 :MeOH, 9:1 after prewashing with 10% Et 3 N in CH 2 Cl 2 ) to yield 2 (0.030 g, 42%) as a yellow solid. 1 H NMR (300 MHz, CDCl 3 ) δ 8.42–8.65 (m, 2H), 7.80–8.08 (m, 2H), 7.37–7.80 (m, 4H), 6.94 (s, 2H), 5.07 (s, 4H), 4.55 (s, 2H), 3.75–3.90 (m, 2H), 3.35–3.40 (m, 2H), 2.10 (s, 6H), 1.01 (s, 9H), 0.17 (s, 6H). HRMS m/z calculated for C 35 H 43 N 3 O 7 Si 645.2949, found 646.2958 ([M+H] + ). Synthesis of 8 Calcium oxide (0.67 g, 12 mmol) was added to a mixture of 4-methoxyphenol (1.49 g, 12.0 mmol) and aqueous formaldehyde (37%, 10 ml) in a plastic tube [67] . The reaction was vortexed in the plastic tube at room temperature in the dark for 5 days and then cooled (5 °C), neutralized with acetic acid and extracted with ether (3 × 40 ml). The organic phase was washed with brine (40 ml), dried over MgSO 4 , filtered and concentrated under reduced pressure. The concentrated filtrate was separated by silica gel chromatography (hexanes to ethyl acetate 7:3) to yield 8 (0.64 g, 67%). 1 H NMR (300 MHz, MeCN-d 3 ) 6.68 (s, 2H), 4.69 (s, 4H), 3.70 (s, 3H) and 13 C NMR (300 MHz, MeCN-d 3 ) 153.58, 148.49, 128.84, 113.17, 62.26, 59.43. HRMS m/z calculated for C 9 H 12 O 4 184.0736, found 184.0740 (M + ); melting point, 100–102 °C. Synthesis of 9 Imidazole (1.70 g, 25.0 mmol) was added to a solution of TBDMSCl (2.40 g, 16.0 mmol) and 8 (0.62 g, 2.7 mmol) in 6 ml of dry DMF under N 2 . The reaction mixture was stirred at room temperature for 16 h, diluted with ether (50 ml) and washed with water (50 ml) and brine (50 ml). The organic phase was dried over MgSO 4 , filtered, concentrated under reduced pressure and subjected to silica gel chromatography (methylene chloride and MeOH 1:19) to yield 9 as a white solid (1.0 g, 60%). 1 H NMR (400 MHz, CDCl 3 ) δ 6.94 (s, 2H), 4.68 (s, 4H), 3.70 (s, 3H), 0.6–1.1 (m, 27H), 0–0.3 (m, 18H). 13 C NMR (500 MHz, CDCl 3 ) 154.6, 141.8, 132.8, 111.1, 60.9, 55.6, 26.3, 18.7, 18.9, −3.1, −5.2. HRMS m/z calculated for C 27 H 54 O 4 Si 3 526.3330, found 526.3318 (M + ). Synthesis of bisQMP3 ( 3 ) Solid ferric chloride (162 mg, 1.00 mmol) was added to a solution of 9 (1.00 g, 1.89 mmol) in acetic anhydride (6 ml) at 0 °C under nitrogen. The reaction mixture was stirred for 2 h and then mixed with ether (80 ml). The organic phase was washed with water (2 × 50 ml) and saturated NaHCO 3 (2 × 50 ml, caution gas release), dried with MgSO 4 and concentrated under reduced pressure. The residue was separated by preparative silica gel TLC (hexane:ethyl acetate, 7:3) to yield bisQMP3 ( 3 ) as a yellowish viscous liquid (0.5 g, 66%). 1 H NMR (400 MHz, CDCl 3 ) 6.85 (s, 2H), 5.03 (s, 4H), 3.79 (s, 3H), 2.11 (s, 6H), 1.06 (s, 9H), 0.18 (s, 6H). 13 C NMR (125 MHz, CDCl 3 ) 171.08, 154.18, 145.04, 128.05, 115.19, 62.03, 55.83, 26.12, 21.12, 18.83, −3.38. HRMS m/z calculated for C 19 H 30 O 6 Si 382.1812, found 382.1809 (M + ). Determining the absorptivity of bisQMP2 (2) and bisQMP3 (3) The extinction coefficient of bisQMP2 (3,600 l/mol cm) was estimated as the sum of extinction coefficients for 9-aminoacridine and the bisQMP parent (bisQMP3) at 297 nm. The extinction coefficient for bisQMP3 (3200, l/mol cm) was measured at 297 nm with serial dilutions. Crosslinking of preannealed duplex DNA Duplex DNA was annealed by combining a labelled 5′-[ 32 P]-oligodeoxynucleotide (50 nCi, 3.0 μM) and its complement (3.3 μM) in MES (10 mM, pH 7), heating the solution rapidly to 90 °C and subsequently cooling slowly to ambient temperature. The bisQMPs were then added as indicated to generate a final solution containing 20% acetonitrile. Aqueous NaF (50 mM) was used to initiate reaction and incubations were maintained under ambient conditions for the specified times. The resulting DNA was either separated directly by denaturing polyacrylamide (20%) gel electrophoresis or treated with hot piperidine (90 °C, 30 min) before gel electrophoresis. Products were quantified by phosphoimagery and reported (%) relative to total labelled DNA. Transfer of crosslinking from intra- to interstrand The desired 5′-[ 32 P]-oligodeoxynucleotide (50 nCi, 3 μM) was treated alternatively with bisQMP1 ( 1 , 12 μM), bisQMP2 ( 2 , 12 μM) or bisQMP3 ( 2 , 4.8 mM) in MES (10 mM, pH 7) and 20% acetonitrile. Reaction was initiated by addition of NaF (50 mM) and maintained at ambient temperature for 24 h. The complementary oligodeoxynucleotide (3.3 μM) was then added to the solution and incubation was continued for the indicated times. Products were separated and analysed as described above. Exchange and migration of crosslinks within duplex DNA As indicated, various acceptor [ 32 P]-oligodeoxynucleotides (50 nCi, 3 μM) were added to a donor duplex of DNA (3.0 μM) containing interstrand crosslinks formed by intra- to interstrand transfer of a bisQM. Samples were incubated under ambient conditions in MES (10 mM, pH 7) and 20% acetonitrile until analysed as describe above using gel electrophoresis and phosphoimagery. How to cite this article: Fakhari, F. and Rokita, S. E. A Walk Along DNA using bipedal migration of a dynamic and covalent crosslinker. Nat. Commun. 5:5591 doi: 10.1038/ncomms6591 (2014).